A primer for academic entrepreneurs on academic-industrial partnerships 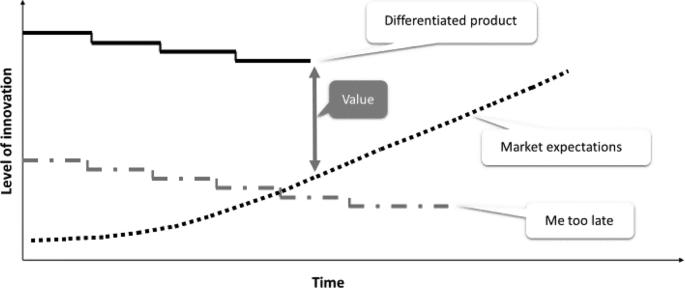Fig. 1: The innovation threshold. Depicts the importance of embarking on a project that will meet market expectations 10 years or more from the time of initiation. The solid back line (top) represents the level of innovation of a differentiated product. The broken gray line (middle) represents the fate of a “me too” drug. The dotted line represents market expectations. For an idea to ultimately reach the marketplace, it will take time; ten years or more for a new drug with costs that vary widely but can run over $2 billion (when the cost of failures is included) [4] . Therefore, one must consider if ten years from an investment, will the product still be valuable, i.e., will it cross the innovation threshold thereby exceeding market expectations through clinical benefit and commercial potential (Fig. 1 )? For example, in the past, the regulatory approval of a new drug with a similar mechanism of action but relatively small improvements in safety and efficacy compared to that of an approved or generic drug might enjoy market success. Today, however, technology assessment agencies such as The National Institute for Health and Care Excellence (NICE) consider whether a new product adds clinical benefit and is cost-effective based on metrics such as gain in quality-adjusted life years (QALYs). Fig. 1: The innovation threshold. Depicts the importance of embarking on a project that will meet market expectations 10 years or more from the time of initiation. The solid back line (top) represents the level of innovation of a differentiated product. The broken gray line (middle) represents the fate of a “me too” drug. The dotted line represents market expectations. Full size image The ability to drive a product from concept to the market begins with great science, scientific leadership, and data that are reproducible and generalizable. At the early stages of discovery, most data packages are incomplete, but the fundamental dataset must be solid. A company will often ask for a material transfer agreement to independently test an asset. One must also consider whether current technologies exist to advance the project or will new ones need to be created. The industrialization of an asset is not a skill possessed by most academic scientists, so the academic entrepreneur is wise to deploy individuals with experience working with the Biopharmaceutical industry, i.e., successful serial entrepreneurs. Faculty members may have less experience with large animal toxicology, manufacturability at scale, regulatory agency guidances, and competitive landscapes. In academic labs, a particular problem can be thoroughly investigated for decades through research grants, talented students, and post-docs. In contrast, a drug discovery campaign needs to be rapidly de-risked so that the resources required to move a product forward can be deployed against the most promising projects within a company’s portfolio. A clear de-risking experiment, i.e., a killer experiment, is one designed to disprove the hypothesis underlying the project. For example, if a lead molecule is purported to selectively inhibit a target enzyme in cancer based on biochemical studies against a large panel of enzymes, a killer experiment could be to test if the drug killed cancer cells in cell lines where the target had been deleted. If the killer experiment fails to support the thesis, this does not necessarily mean that given enough time and money that the program will never succeed. Rather, there is an opportunity cost in continuing to pursue this idea rather than investing in others. It is difficult to assess the value of an early project. Industry calculates the probability of technical and regulatory success (PTRS) and uses this calculation to approximate the net present value (NPV) of an executed deal. Since early projects may have a negative risk-adjusted net present value (eNPV), an entrepreneur might be disappointed by the terms. Therefore, it is important that deal terms are carefully developed, clearly explained, and are viewed as fair. Important considerations include fair market value determined by analyzing recent, similar types of deal constructs, i.e., comparables, intellectual property filings, and approvals. Companies will want to know the costs to reach the next decision point, for example, the resources required to conduct the killer experiment. Deals will often be constructed with an upfront payment and research support to get to this milestone. The construct will then be backloaded, i.e., payments for later successes, such as the declaration of a clinical candidate, Investigational New Drug (IND) Application or New Drug Application (NDA) filing or approval, the first patient in a Phase 1 clinical study, Phase 2 proof of concept, and entry into a Phase 3 registrational study. Financial terms may also include sales milestones and royalties. The buyer will then generate a non-binding term sheet (NBTS), which is a preliminary construct of what and how the company would be willing to pay. A NBTS is sometimes required by originators before allowing the potential partner to proceed to a deeper level of due diligence. The NBTS should never be used as a fishing expedition to gain inside or competitive information, but rather it is a good-faith starting point for negotiations. There are also times when an equity investment in a newly formed company (NewCo) would be beneficial to the partners. Depending on where the company or asset is in its evolution, a valuation is created. It is important for originators to understand the implications of an investment in the context of pre-money and post-money valuations. Pre-money is how investors value the company today, i.e., prior to an additional investment. Post money is the valuation after adding the new investment. For example, if an originator raises $2 million at a $6 million pre-money valuation, the post-money valuation is $8 million. That $2 million invested in a company valued post-money at $8 million gives the investor 25% ownership of the company [5] . Companies may ask for rights. These include the right of first refusal, i.e., the right to match an offer from a third party, right of first negotiation, i.e., the right to negotiate an offer before the asset is sold to someone else, or a pre-negotiated option price to execute a deal later at an upfront agreed-upon price. If the intellectual property exists, the company may also ask for rights to a sub-license. A company may ask for a period of exclusivity, which has both risks (exclusion of others) and benefits (a dedicated potential buyer) for the originator. Finally, there are several intangibles. For example, as in any partnership, there should be cultural compatibility. In essence, the chemistry between the originator and the investor can be a deciding factor. Above all, the opportunity for a partnership between academia and industry provides originators with the opportunity to see their work become lifesaving products for millions of people around the world, a shared goal with industry colleagues. In conclusion, partnerships between academia and industry are essential components of the innovation pipeline, and a better understanding of the criteria used to assess these collaborations can help to streamline the process.